Epidemiology ofPlasmodium malariaeandPlasmodium ovalespp. in Kinshasa Province, Democratic Republic of Congo Reports suggest non-falciparum species are an underappreciated cause of malaria in sub-Saharan Africa but their epidemiology is ill-defined, particularly in highly malaria-endemic regions. We estimated incidence and prevalence of PCR-confirmed non-falciparum and Plasmodium falciparum malaria infections within a longitudinal study conducted in Kinshasa, Democratic Republic of Congo (DRC) between 2015-2017. Children and adults were sampled at biannual household surveys and routine clinic visits. Among 9,089 samples from 1,565 participants, incidences of P. malariae, P. ovale spp., and P. falciparum infections by 1-year were 7.8% (95% CI: 6.4%-9.1%), 4.8% (95% CI: 3.7%-5.9%) and 57.5% (95% CI: 54.4%-60.5%), respectively. Non-falciparum prevalences were higher in school-age children, rural and peri-urban sites, and P. falciparum co-infections. P. falciparum remains the primary driver of malaria in the DRC, though non-falciparum species also pose an infection risk. As P. falciparum interventions gain traction in high-burden settings, continued surveillance and improved understanding of non-falciparum infections are warranted. Reports of non-falciparum malaria caused by Plasmodium malariae and Plasmodium ovale spp. have increased across sub-Saharan Africa, where more than 95% of global malaria cases and deaths occur [1] . Plasmodium falciparum is the primary cause of malaria morbidity and mortality in the region. However, molecular surveys have confirmed co-circulating non-falciparum species, and suggest a rise in prevalence in regions where P. falciparum has declined [2] , [3] , [4] , [5] , [6] . Despite this, our understanding of infection risk and clinical burden posed by non-falciparum species is limited, particularly within regions of high P. falciparum transmission. The Democratic Republic of Congo (DRC) is one of 11 malaria “High Burden, High Impact” countries designated by the World Health Organization (WHO) [7] , indicating a critical need to understand the full landscape of malaria transmission and infection in the country. The DRC harbors the second highest burden of malaria worldwide, accounting for 12% of global malaria cases and 13% of malaria-related deaths as of 2020 [1] . Transmission is largely stable and perennial throughout the country, with an estimated 97% of the population living in high malaria transmission regions for eight or more months per year [8] , [9] , [10] . While the majority of the country is characterized as hyper- and holo-endemic for malaria [8] , [9] , [11] , transmission can vary within and across provinces due to environmental and geographical factors such as urbanicity, population density, land use, temperature, and rainfall [10] , [12] . In Kinshasa Province, home to the capital city of Kinshasa, malaria transmission is lower within the central urban areas, and increases in the outer peri-urban and rural zones [10] . While P. falciparum accounts for the vast majority of infections in the DRC, P. malariae and P. ovale spp. have been documented at low-level prevalences [8] , [13] , [14] , [15] ; however, their epidemiology and clinical impact remains poorly understood. Existing non-falciparum prevalence estimates were largely derived from cross-sectional studies, limiting risk assessment, or focused on a singular age group or symptomatic status, which restricts broader generalizability [13] , [15] , [16] , [17] , [18] , [19] , [20] , [21] . The absence of reliable field diagnostics for these less-common infections complicates surveillance efforts and case management. Gold-standard microscopy methods can detect non-falciparum parasites, but insufficient training and specialization ultimately limits the sensitivity and specificity for non-falciparum infections [22] . Widely-used malaria rapid diagnostic tests (RDTs) in Africa cannot distinguish P. malariae or P. ovale spp. infections. While most RDTs detect P. falciparum- specific histidine-rich protein 2 (HRP2), and some also detect Plasmodium lactate dehydrogenase (LDH), no P. malariae and P. ovale spp. - specific RDTs are currently available. Further, clinical diagnosis of a non-falciparum infection is not feasible in the absence of symptoms attributed specifically to P. malariae or P. ovale spp. These infections are complicated to detect in malaria-endemic regions such as the DRC where P. falciparum co-infection is common, making it difficult to distinguish symptoms caused specifically by these non-falciparum species. P. malariae infections have been associated with acute febrile illness and anemia [23] , [24] , [25] as well as chronic nephrotic syndrome [26] , [27] . P. ovale spp. infections commonly result in low morbidity, although severe complications have been documented in case reports [28] , [29] . The clinical relevance of P. falciparum co-infection with non-falciparum species is also unclear, with posited suppressive effects observed in one study [4] , while another detected severe malaria among mixed-infections [24] . These diagnostic challenges are exacerbated by low parasite densities characteristic of non-falciparum infections, which require the use of sensitive laboratory assays that are not suitable for routine field use. P. malariae and P. ovale spp. infections have occasionally been dismissed as rare infections that are not clinically impactful in high-burden countries like the DRC. However, improved characterization of their epidemiology and clinical implications is needed to determine their proper place in malaria programmatic and surveillance efforts. Leveraging a 34-month longitudinal cohort study conducted across diverse sites in Kinshasa Province, DRC, we sought to determine the epidemiology of P. malariae and P. ovale spp. infections in the context of high P. falciparum transmission. We performed high-throughput, real-time polymerase chain reaction (PCR) on samples collected from both asymptomatic and symptomatic participants of all ages as part of a large longitudinal study of non-falciparum malaria infection. We estimated incidence, associated factors, and clinical features associated with P. malariae and P. ovale spp. infections over time, and as compared to P. falciparum infections. Study population A total of 1591 individuals were enrolled in the parent cohort across 242 households and seven sites in Kinshasa Province, DRC. Among these, 1565 (98.4%) participants had a baseline dried blood spot (DBS) sample available for analysis and were included in this study, contributing 5682 total survey visits. Participant follow-up by analysis population is displayed in Fig. 1 . In the main survey population, 76% of participants completed all three study follow-ups; loss-to-follow-up differed by regional health area, with a higher proportion observed in peri-urban (28%, n = 143) and urban (30%, n = 116) health areas compared to rural (18%, n = 116). Sixty-seven percent ( n = 1050) of those in the main survey population also had ≥1 symptomatic clinic visit during the 34-month passive follow-up period and were included in the clinic-based analysis, comprising 218 (90.1%) of the 242 enrolled households. Participants in the clinic subpopulation had 3407 total clinic visits, with a median (interquartile range [IQR]; min-max) of 2 (1−4; 1−19) visits per person and 11 (5−22; 1−74) per household. Fig. 1: Study population. The study population comprised 1565 enrolled participants who had a DBS sample at the baseline visit. Participants without a baseline DBS were excluded from analyses. Participant loss-to-follow-up among the survey-based population is shown, with 76% completing all three follow-up visits. Sixty-seven percent of participants in the survey population visited a study health clinic at least once during follow-up, comprising the clinic-based subpopulation. Study health clinic visit frequency across the full study period is shown. The total population encompassed all survey and clinic-based study visits. DBS dried blood spot, FU follow-up. 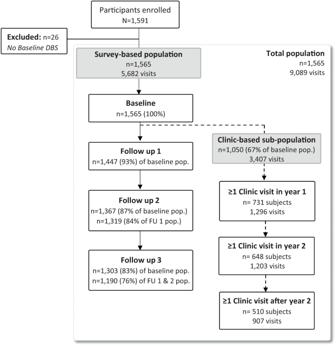Fig. 1: Study population. The study population comprised 1565 enrolled participants who had a DBS sample at the baseline visit. Participants without a baseline DBS were excluded from analyses. Participant loss-to-follow-up among the survey-based population is shown, with 76% completing all three follow-up visits. Sixty-seven percent of participants in the survey population visited a study health clinic at least once during follow-up, comprising the clinic-based subpopulation. Study health clinic visit frequency across the full study period is shown. The total population encompassed all survey and clinic-based study visits. DBS dried blood spot, FU follow-up. Full size image Baseline demographic and clinical characteristics for the survey population are summarized in Table 1 . The median (IQR) age of participants at baseline was 14 (6−31) years, with 19% of participants aged <5 years, and 32% school-aged (between 5 and 14 years). The majority of participants in the survey population were female (55%), and 42% were living in rural sites. Approximately 73% of the population lived in a household with at least one bed net, although only 45% reported sleeping under a bed net. Twenty-four percent of participants self-reported having a fever in the week prior to baseline, 25% reported experiencing malaria symptoms in the prior 6 months and taking antimalarials, and 27% of participants had a positive malaria RDT at the baseline survey. Table 1 Baseline participant characteristics by species –survey population Full size table Baseline characteristics were similar between those also included in the symptomatic clinic subpopulation, and the full survey population (Supplementary Table 1 ). The median (IQR) age of participants in the clinic subpopulation was 12 (5–30) years, with 22% aged <5 years, and 34% school-aged (5–14 years). 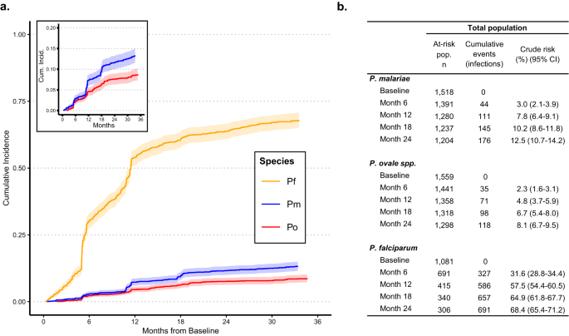Fig. 2: Cumulative incidence ofPlasmodiuminfections across 34-months of follow-up in the total study population. aCumulative incidence curves depict time to the first detectedP. malariae(blue),P. ovale(red), andP. falciparum(yellow) infections among participants negative for eachPlasmodiumspecies infection at baseline. Shading depicts 95% CIs around cumulative incidence estimates. Incidence curves increase in a step-wise fashion at follow-up survey timepoints due to participant-wide screening and case detection, whereas gradual slopes in between survey timepoints indicate additional incident events detected through symptomatic presentation to clinics.bCrude risks of incident infections among the total population shown in Fig.2a, by malaria species. Time to the first incident infection since baseline. CI confidence interval, PfPlasmodium falciparum,PmPlasmodium malariae,PoPlasmodium ovalespp. There was also a higher proportion of women (56%) than men in the clinic subpopulation, and higher proportions of participants living in rural (22%) or peri-urban (32%) sites compared to urban sites (46%), as in the broader survey population (Supplementary Table 2 ). 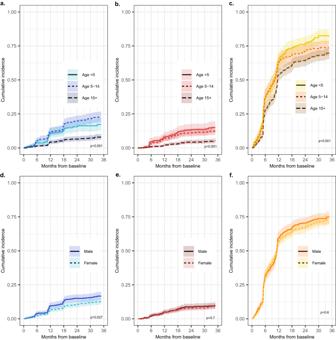Fig. 3: Cumulative incidence curves stratified by participant characteristics. Cumulative incidence of first infection stratified by age at baseline, forP. malariae(n= 1518; <5 years:n= 296, 5–14 years:n= 470; 15+ years:n= 752 at risk at baseline) in blue (a),P. ovalespp. (n= 1557; <5 years:n= 301, 5–14 years:n= 498; 15+ years:n= 758 at risk at baseline) in red (b), andP. falciparum(n= 1081; <5 years:n= 238, 5–14 years:n= 260; 15+ years:n= 583 at risk at baseline) in yellow (c). Cumulative incidence of first infection stratified by sex, forP. malariae(n= 1518; female:n= 840, male:n= 678 at risk at baseline) in blue (d),P. ovalespp. (n= 1559; female:n= 858, male:n= 701 at risk at baseline) in red (e), andP. falciparum(n= 1081; female:n= 618 male:n= 463 at risk at baseline) in yellow (f).p-values are calculated from log-rank testing. Shading depicts 95% CIs around incidence estimates. CI confidence interval. 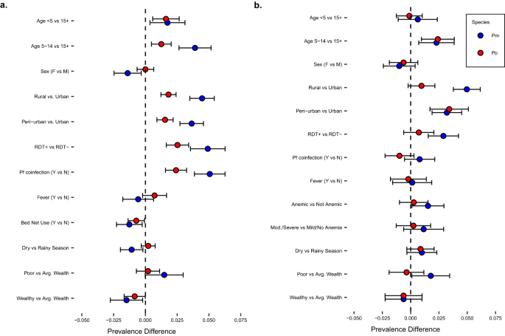Fig. 4: Factors associated withP. malariaeandP. ovalespp. infection prevalence, stratified by survey vs. clinic-based population. aFactors associated withP. malariae(blue) andP. ovale(red) infection prevalences at survey visits (baseline and three follow-up surveys).bFactors associated withP. malariae(blue) andP. ovale(red) prevalences at symptomatic clinic visits across follow-up (i.e., symptomatic cases). Error bars represent 95% CIs around unadjusted prevalence difference measures; numerical values of prevalence differences and 95% CIs are listed in Supplementary Tables8and9.n= 5659 biologically independent samples in the survey population (a), andn= 3349 in the clinic-based population (b). Factors associated with non-falciparum infection prevalences compared toP. falciparuminfection are depicted in Supplemental Fig.2. CI confidence interval, PfPlasmodium falciparum,PmPlasmodium malariae,PoPlasmodium ovalespp., RDT rapid diagnostic test. Participant characteristics across follow-up visits are summarized in Supplementary Table 3 and Supplementary Table 4 . Overall, 97.0% ( n = 1518) and 99.6% ( n = 1559) of participants were PCR-negative for a P. malariae and P. ovale spp. infection at baseline, respectively; 69.1% ( n = 1081) were PCR-negative for a P. falciparum infection at baseline. These PCR-negative participants comprised at-risk populations for malaria incidence estimation. Incidence of non-falciparum malaria infections The estimated 1-year cumulative incidences of P. malariae and P. ovale spp. infections were 7.8% (95% CI: 6.4%–9.1%) and 4.8% (95% CI: 3.7%–5.9%), respectively, encompassing the first incident infections detected at survey or clinic visits. Comparatively, 57.5% (95% CI: 54.4%–60.5%) of at-risk participants acquired a P. falciparum infection by 1-year (Fig. 2 ). Risk of P. malariae and P. ovale spp. was similar within the first year of follow-up, but appears to increase at, and following, the second study follow-up visit around 1-year from baseline, after which the risk of a P. malariae infection surpassed that of P. ovale spp. Time to the first detected infection was faster for P. falciparum than P. malariae or P. ovale infections throughout the whole study period, with at least half of the total at-risk population experiencing a P. falciparum malaria infection by 12 months from baseline. Step-wise increases in incidence depicted in Fig. 2 represent infections detected at periodic household surveys; symptomatic infections detected through passive, clinic-based surveillance filled in gaps between surveys, as indicated by steady inclines between step-ups. The 1-year cumulative incidences of first P. malariae and P. ovale spp. infections detected only at active surveillance household surveys were approximately 4.9% (95% CI: 3.7%–6.0%) and 3.4% (95% CI: 2.4%–4.3%), respectively, including single- and mixed-species infections, whereas the cumulative incidence of a P. falciparum infection by 1-year was 42.8% (95% CI: 39.6%–45.8%) within the survey population (Table 2 ). Fig. 2: Cumulative incidence of Plasmodium infections across 34-months of follow-up in the total study population. a Cumulative incidence curves depict time to the first detected P. malariae (blue), P. ovale (red), and P. falciparum (yellow) infections among participants negative for each Plasmodium species infection at baseline. Shading depicts 95% CIs around cumulative incidence estimates. Incidence curves increase in a step-wise fashion at follow-up survey timepoints due to participant-wide screening and case detection, whereas gradual slopes in between survey timepoints indicate additional incident events detected through symptomatic presentation to clinics. b Crude risks of incident infections among the total population shown in Fig. 2a , by malaria species. Time to the first incident infection since baseline. CI confidence interval, Pf Plasmodium falciparum, Pm Plasmodium malariae, Po Plasmodium ovale spp. Full size image Table 2 Incidence of infection during household survey visits and symptomatic clinic visits, by Plasmodium species Full size table Cumulative incidences of first P. malariae, P. ovale spp., and P. falciparum infections stratified by age and sex are depicted in Fig. 3 . Within the total study population, cumulative incidences of first P. malariae and P. ovale spp. infection were higher among children <5 and school-aged children 5–14 years old compared to participants aged ≥15 years ( Pm : p < 0.001; Po : p < 0.001). Time to the first detected P. ovale spp. infection was similar between children <5 and 5–14 years throughout follow-up, whereas school-aged children 5–14 years old experienced a faster time to P. malariae infection, particularly towards the end of follow-up driven by symptomatic clinic-based infections. The cumulative incidence of first P. falciparum infection was also higher among children <5 and 5–14 years old, compared to adults aged ≥15, although P. falciparum incidences were high (≥50%) across all age categories by 1-year ( p < 0.001). No differences in the cumulative incidence of P. ovale spp. and P. falciparum infection by sex were detected ( p = 0.73 and p = 0.62, respectively), although P. malariae infection incidence was higher among males than females ( p = 0.03). Fig. 3: Cumulative incidence curves stratified by participant characteristics. Cumulative incidence of first infection stratified by age at baseline, for P. malariae ( n = 1518; <5 years: n = 296, 5–14 years: n = 470; 15+ years: n = 752 at risk at baseline) in blue ( a ), P. ovale spp. ( n = 1557; <5 years: n = 301, 5–14 years: n = 498; 15+ years: n = 758 at risk at baseline) in red ( b ), and P. falciparum ( n = 1081; <5 years: n = 238, 5–14 years: n = 260; 15+ years: n = 583 at risk at baseline) in yellow ( c ). Cumulative incidence of first infection stratified by sex, for P. malariae ( n = 1518; female: n = 840, male: n = 678 at risk at baseline) in blue ( d ), P. ovale spp. ( n = 1559; female: n = 858, male: n = 701 at risk at baseline) in red ( e ), and P. falciparum ( n = 1081; female: n = 618 male: n = 463 at risk at baseline) in yellow ( f ). p -values are calculated from log-rank testing. Shading depicts 95% CIs around incidence estimates. CI confidence interval. Full size image Prevalence of non-falciparum and P. falciparum infections Among 1565 participants across all baseline and follow-up household surveys in the approximately 2-year active surveillance period, 159 (10.2%) participants had 186 PCR-confirmed P. malariae infections, 70 (4.5%) participants had 78 P. ovale spp. infections, and 990 (63.3%) participants had 1976 P. falciparum infections detected. Of all 5682 tested samples collected from these participants across household follow-up surveys, 3.3% (95% CI: 2.8%–3.8%) were PCR-positive for a P. malariae infection, 1.4% (95% CI: 1.1%–1.7%) for a P. ovale spp. infection, and 34.9% (95% CI: 33.2%–36.5%) for a P. falciparum infection. The majority of P. malariae and P. ovale spp. infections in the survey-based population were mixed-species ( P. malariae: 73.7% [ n = 137/186]; P. ovale spp. : 78.2% [ n = 61/78]), and were predominately co-infected with P. falciparum . In contrast, the vast majority of P. falciparum infections were single-species (90.5%; n = 1788/1976). P. malariae prevalence across household survey visits remained steady throughout active follow-up, fluctuating between 3.0% at baseline, 2.4% at follow-up 1, 4.1% at follow-up 2, and 3.7% at the final household survey ( p = 0.06; Supplementary Table 3 ). Similarly, P. ovale spp. prevalence remained relatively low across follow-up, with 0.4% of the population infected with P. ovale spp. at baseline, increasing to 1.9% and 2.0% at follow-ups 1 and 2, and ending at a 1.4% prevalence by the final follow-up ( p < 0.01; Supplementary Table 3 ). P. falciparum prevalence increased slightly over time, with the highest prevalence (39.6%) detected at the second follow-up visit in the rainy season ( p < 0.01; Supplementary Table 3 ). Similar prevalences to those detected in the survey population were observed among the symptomatic clinic subpopulation, despite longer clinic-based follow-up. Among 1050 participants who visited study clinics in the approximately 3-year clinic-based surveillance follow-up period, a total of 120 (11.4%) patients had 135 P. malariae infections detected, and 80 (7.6%) patients had 95 P. ovale spp. infections detected. However, prevalence of P. falciparum was higher in symptomatic clinic patients compared to the survey population, with 789 (75.1%) patients having 2009 P. falciparum infections. From the clinic subpopulation, 4.0% (95% CI: 3.3%–4.7%) of all 3407 tested clinic samples across the clinic-based surveillance follow-up period were PCR-positive for a P. malariae infection, 2.8% (95% CI: 2.2%–3.4%) for a P. ovale spp. infection, and 58.7% (95% CI: 56.5%–60.8%) for a P. falciparum infection. The timeline of all P. malariae and P. ovale spp. infections by participant throughout the full study is depicted in Supplementary Fig. 1 . Multiple non-falciparum infections of the same species were detected over time at survey or clinic-based surveillance visits in 23.5% ( n = 58/247) of all participants who had a P. malariae infection, and in 21.6% ( n = 30/139) of those who had a P. ovale spp. infection during the 34-month study period. Three participants each had a P. malariae infection detected 4 times throughout follow-up. In comparison, P. falciparum infections re-occurred frequently, with 75.2% ( n = 914/1216) of those who had a P. falciparum infection having more than one during follow-up, and 22.4% ( n = 272/1216) having ≥5 P. falciparum infections detected during the 34-month study period. Children had non-falciparum infections more frequently than adults. Prevalence of P. malariae infection in the survey-based population was highest among school-aged children aged 5–14 years at 5.6% (95% CI: 4.4%–6.7%), though still low overall, followed by children <5 years (3.4% [95% CI: 2.1%–4.7%]), and lowest among those aged ≥15 (1.7% [95% CI: 1.2%–2.2%]). Conversely, children <5 years experienced a slightly higher prevalence of P. ovale spp. infection compared to school-aged children (2.3% [95% CI: 1.3%–3.3%] vs. 1.9% [95% CI: 1.2%–2.7%]), although prevalences across both age groups were low overall, and lower than P. malariae prevalence in these age groups; 0.7% (95% CI: 0.4%–1.0%) of adults ≥15 years had a P. ovale spp. infection at study survey visits. Factors associated with the prevalence of P. malariae and P. ovale spp. infections are shown in Fig. 4 (and Supplementary Tables 8 and 9 ), and contrasted with P. falciparum prevalence differences (PD) in Supplementary Fig. 2 . Within the survey-based population, P. falciparum coinfection was associated with an increased prevalence of both P. malariae (PD 0.05 [95% CI: 0.04–0.06]) and P. ovale spp. (PD: 0.02 [95% CI: 0.02–0.03]) infections. In comparison to those with average wealth, higher wealth was associated with a decreased prevalence of P. malariae (PD: -0.01 [95% CI: -0.03 to -0.002]) and P. ovale spp. (PD: -0.01 [95% CI: -0.02 to -0.00]) infection. School-aged children 5–14 years old were associated with a higher prevalence of P. malariae (PD: 0.04 [95% CI: 0.03–0.05]) and P. ovale spp. (PD: 0.01 [95% CI: 0.005–0.02]), infection as compared to participants 15 and older and also as compared to children aged <5 for P. malariae (PD: 0.02 [95% CI: 0.005–0.04]). Additionally, both P. malariae and P. ovale spp. infection prevalences were higher among participants living in rural ( Pm: PD: 0.04 [95% CI: 0.03–0.05]; Po : PD: 0.02 [95% CI: 0.01–0.02]) and peri-urban ( Pm: PD: 0.04 [95% CI: 0.03–0.05]; Po: PD: 0.02 [95% CI: 0.01–0.02]) sites as compared to an urban setting. Fig. 4: Factors associated with P. malariae and P. ovale spp. infection prevalence, stratified by survey vs. clinic-based population. a Factors associated with P. malariae (blue) and P. ovale (red) infection prevalences at survey visits (baseline and three follow-up surveys). b Factors associated with P. malariae (blue) and P. ovale (red) prevalences at symptomatic clinic visits across follow-up (i.e., symptomatic cases). Error bars represent 95% CIs around unadjusted prevalence difference measures; numerical values of prevalence differences and 95% CIs are listed in Supplementary Tables 8 and 9 . n = 5659 biologically independent samples in the survey population ( a ), and n = 3349 in the clinic-based population ( b ). Factors associated with non-falciparum infection prevalences compared to P. falciparum infection are depicted in Supplemental Fig. 2 . CI confidence interval, Pf Plasmodium falciparum, Pm Plasmodium malariae, Po Plasmodium ovale spp., RDT rapid diagnostic test. Full size image Similarly, in the clinic-based analysis, school-aged children were also associated with an increased prevalence of P. malariae (PD: 0.02 [95% CI: 0.01–0.04]) and P. ovale spp. (PD: 0.02; [95% CI: 0.01– 0.04]), infections, compared to adults ≥15 and older; however, no differences in prevalence of P. malariae and P. ovale spp. were observed between children <5 years and adults ≥15 and older in this symptomatic population ( Pm : PD: 0.01 [95% CI: -0.01–0.02]; Po : PD: -0.001 [95% CI: -0.01–0.01]). In contrast to the survey population, no associations were observed with P. falciparum co-infection for either non-falciparum species in the clinic-based analysis ( Pm : PD: 0.01 [95% CI: -0.01–0.02]; Po : PD: -0.01 [95% CI: -0.02–0.003]). P. malariae infection prevalences were higher among rural (PD: 0.05 [95% CI: 0.04–0.06]) and peri-urban (PD: 0.03 [95% CI: 0.02–0.05]) sites as compared to urban in the clinic-based analysis, whereas no difference in P. ovale spp. prevalence was observed between rural and urban settings among symptomatic participants (PD: 0.01 [95% CI: -0.002–0.02]). Prevalence of self-reported fever in the week prior to the survey visit was similar for P. malariae (PD: -0.006 [95% CI:-0.018–0.006]) and P. ovale spp. infections (PD: 0.007 [95% CI: -0.002–0.017]), as compared to no species-specific malaria infection among the survey population (Fig. 4 ). In the symptomatic clinic subpopulation, concurrent anemia of any severity was associated with P. malariae infection prevalence (PD: 0.015 [95% CI: 0.001–0.029]), although associations were no longer significant when stratifying by anemia severity, comparing moderate-to-severe cases vs. mild or no anemia for P. malariae (PD: 0.012 [95% CI: -0.006–0.029]), or for P. ovale spp. (PD: 0.002 [95% CI:-0.013–0.018]. Differences in parasite densities by species mixed infections Estimated median (IQR) parasite densities were low (<50 parasites [p]/µL) among all non-falciparum infections in the study ( P. malariae : 25.7 [7.7–119] p/µL, n = 307; P. ovale : 10.2 [2.7–47.4] p/µL, n = 164), while median (IQR) P. falciparum parasite densities in the total population were higher at 267 p/µL (18.8–4526 p/µL, n = 3730). Non-falciparum parasite densities remained low when stratified by survey population ( P. malariae : 22.4 [8.5–72.2] p/µL, n = 175; P. ovale spp. : 5.8 [2.0–28.0] p/µL, n = 71), vs. symptomatic clinic sub-population ( P. malariae : 36.5 [4.7–182] p/µL, n = 132; P. ovale : 17.7 [4.6–65.8] p/µL, n = 93). Parasite density distributions were slightly higher among P. malariae infections than P. ovale spp. infections. We did not detect any differences in estimated P. malariae or P. ovale spp. parasite density distributions between mixed- vs. single-species P. malariae or P. ovale spp. infections in the total population ( P. malariae: p = 0.071; P. ovale : p = 0.465), or across specific population types. 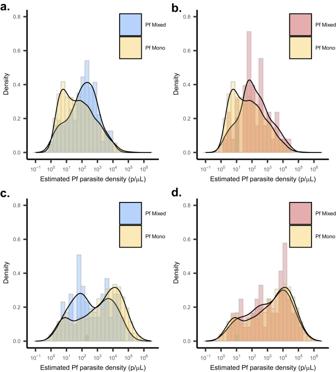Fig. 5: Distributions ofP. falciparumparasitemia by type of non-falciparum mixed infection vs.P. falciparummono infections, stratified by population. Household survey-based results forP. falciparumparasitemia distributions comparingP. falciparummono infections (n= 3418) in yellow vs. co-infection with (a)P. malariae(n= 206) in blue and (b)P. ovalespp. (n= 96) in red. Clinic sub-populationP. falciparumparasitemia distributions comparingP. falciparummono infections (n= 1834) in yellow vs. co-infection with (c)P. malariae(n= 84) in blue and (d)P. ovalespp. (n= 47) in red. Density distributions are displayed to illustrate trends in overall distributions accounting for variation in sample sizes across groups. PfPlasmodium falciparum. Parasite densities are summarized in Supplementary Table 5 ; samples rehydrated during molecular analysis were excluded from analysis ( n = 591 total). Interestingly, differences in the distribution of P. falciparum parasite densities were observed between single-species P. falciparum infections vs. mixed-species infections with P. malariae , but not mixed P. ovale spp. in the clinic subpopulation (Fig. 5 ). A higher median (IQR) P. falciparum parasite density was observed within mixed P. falciparum- P. malariae co-infections (127 [25–496] p/µL, n = 122; vs. 47 [7.4–311] p/µL, n = 1584; p = 0.001) and P. falciparum- P. ovale co-infections (122 [42.2–486] p/µL, n = 49; vs. 47 [7.4–311] p/µL, n = 1584; p = 0.01) as compared to single-species P. falciparum infections among the survey population. However, a lower median P. falciparum parasite density was observed within mixed P. falciparum- P. malariae infections ( n = 84) compared to P. falciparum single-species infections ( n = 1834) in the clinic-based sub-population (288 [57–4319] p/µL vs. 2897 [127–18,058 p/µL; p < 0.001); this association was not observed for P. falciparum- P. ovale co-infections (1710 [165–13,082] p/µL, n = 47; vs. 2897 [127–18,058] p/µL; p = 0.596), although the sample size for mixed P. falciparum-P. ovale co-infections was smaller than for single-species P. falciparum infections. Fig. 5: Distributions of P. falciparum parasitemia by type of non-falciparum mixed infection vs. P. falciparum mono infections, stratified by population. Household survey-based results for P. falciparum parasitemia distributions comparing P. falciparum mono infections ( n = 3418) in yellow vs. co-infection with ( a ) P. malariae ( n = 206) in blue and ( b ) P. ovale spp. ( n = 96) in red. Clinic sub-population P. falciparum parasitemia distributions comparing P. falciparum mono infections ( n = 1834) in yellow vs. co-infection with ( c ) P. malariae ( n = 84) in blue and ( d ) P. ovale spp. ( n = 47) in red. Density distributions are displayed to illustrate trends in overall distributions accounting for variation in sample sizes across groups. Pf Plasmodium falciparum . Full size image P. malariae and P. ovale spp. malaria infections were detected across all sites included in this study, affecting children and adults across a range of P. falciparum transmission intensities in Kinshasa Province, DRC. In the largest longitudinal study of non-falciparum malaria conducted to-date in the DRC, we observed an 8% cumulative incidence of first P. malariae infection and 5% incidence of first P. ovale spp. infection within 1-year, including both asymptomatic and symptomatic infections. Over half of the study population in this high malaria-burdened country experienced an incident P. falciparum infection within 1-year from baseline, confirming the central importance of P. falciparum in the DRC. Over 70% of the non-falciparum infections detected occurred as co-infections with P. falciparum . Though P. falciparum was the dominant species, we detected a considerable risk of infection by a non-falciparum species, particularly for children under 15 years of age. These findings underscore the need to consider these neglected species in areas of high P. falciparum transmission. Ten percent of household survey participants had at least one P. malariae infection during the study, and 5% had at least one P. ovale spp. infection, including both mixed- and single-species infections. Similar prevalences were observed among symptomatic individuals during clinic-based surveillance. Prevalences generally align with previous estimates of non-falciparum infections in the DRC derived from cross-sectional studies [13] , [15] , [16] , [17] , [18] , [19] , [20] , [21] , [30] . Infection prevalences were stable across the 34-month follow-up, differing from recent studies in neighboring countries, which have detected increases in P. malariae and P. ovale infection prevalence over time, particularly as P. falciparum prevalences have started to decline [3] , [4] , [6] . The high proportion of participants with P. malariae who had infection detected more than once during the study (24%) is notable given that this parasite can persist in the blood at low parasite density for long periods of time [25] , [31] , [32] . Chronic P. malariae infection may be associated with deleterious clinical outcomes, such as severe anemia and chronic nephrotic syndrome [24] , [25] , [33] . Though we could not distinguish whether multiple P. malariae infections detected in an individual were due to chronic occurrences or acute reinfection events, future work may allow us to differentiate these infection types. Such work is necessary given a dearth of evidence on the commonality of chronic P. malariae infection, as well as reinfection rates for non-falciparum species in regions highly endemic for P. falciparum . Populations experiencing a P. malariae or P. ovale spp. infection were similar but not identical to those infected with P. falciparum . School-aged children were found to have higher prevalences of P. malariae infection than children under 5 years of age, following similar age-related infection associations with P. falciparum that have been previously established in the region [34] , [35] . Dissimilar from P. falciparum infection patterns, symptomatic children under 5 had comparable P. malariae infection prevalences as those experienced by symptomatic adults aged 15 and older. All Plasmodium species were generally more common in rural and peri-urban sites, and less common in the wealthiest households. We observed a crude association between P. malariae infection prevalence and anemia of any severity in the symptomatic clinic subpopulation, which translated to a 1.5% absolute increase in prevalence compared to those without anemia. Although, this association was no longer significant when stratifying by anemia severity, and was not detected among P. ovale spp. infections in this study. Similarly, no association between non-falciparum infections and fever was detected within the survey- or clinic-based analyses, though misclassification of fever is possible if fever-reducing medicines were taken prior to clinic visits, as data on use of fever-reducing medicines was not captured in this study. Prior studies have posited a protective effect of co-infection with P. falciparum and non-falciparum species on reduced clinical outcomes, compared to single-species P. falciparum infections [36] , [37] , although this has not been consistently observed across studies [38] , [39] . We did not assess causal effects of non-falciparum infection on clinical outcomes in our study due to the limited number of positive samples (though no crude associations were detected in the unadjusted models), including the possibility of attenuated P. falciparum symptoms due to mixed-species infection. Interestingly, P. falciparum parasite densities were higher in mixed infections with P. malariae or P. ovale spp. in the household survey-based, but not clinic-based, analysis. One possible explanation is that P. falciparum increases its virulence to compete with non-falciparum species within the asymptomatic host, though this is an unproven hypothesis that our data are insufficient to evaluate. Non-falciparum parasite densities observed in this study were low, as is characteristic of P. malariae and P. ovale spp. infections. We did not identify any difference in non-falciparum parasite density between mixed and single-species non-falciparum infections. Our incidence and prevalence estimates should be considered lower bounds of the true incidence and prevalence in the study catchment area owing to several limitations of the study. First, the biannual frequency of household surveys missed infections that occurred and resolved between study visits. Also, while the longitudinal design provides helpful insight into risk of infection surrounding these species, the study’s sample size and duration of the study likely limited our ability to detect changes in the prevalence of these less-common species over time in the DRC, where gains in malaria control have not been achieved as in other settings. Second, while loss to follow-up was low overall in the study, missed study visits, early loss to follow-up, and differences in study clinic attendance across sites may have introduced selection bias into the study. Participants may have elected to visit alternative health facilities for malaria care instead of presenting to study clinics. However, all participants were eligible for free malaria treatment at study clinics to encourage use of the study facilities for care and increase representativeness of the clinic subpopulation to the overall study population. Third, our duplex PCR assay detected low density infections with a limit of detection between 1 and 10 p/µL, but would likely miss infections of parasite densities below this range, which are known to occur with P. malariae and P. ovale species. Fourth, some misclassification of seasonality may be present, as local classifications for seasonality by month, rather than rainfall amounts, were used to define rainy seasons. Finally, our observational study design is not immune to the risk of unmeasured confounding, although no causal relationships were assessed in this study. Associated factors depict crude associations only, and while the sample size was relatively large, findings may be affected by the lower prevalence of P. malariae and P. ovale events. This study provides insight into the epidemiology of P. malariae and P. ovale species in a region heavily affected by P. falciparum malaria. Though less common and impactful than P. falciparum, P. malariae and P. ovale spp. infections occurred across all sites and subpopulations, and were often detected within symptomatic clinic-based cases in this large longitudinal study in the DRC. Malaria research and control efforts focused on P. falciparum should also consider these neglected species, particularly in school-aged children and rural communities as part of efforts to progress toward malaria elimination. Study design This study leverages data and samples collected during a longitudinal cohort study of malaria transmission across seven sites within three health areas of varying urbanicity and malaria endemicity in Kinshasa Province, DRC between 2015 and 2017. Detailed methods for site and household sampling have been previously described [34] , [40] . In brief, households were selected at random within the seven chosen villages, and household members were enrolled into the study following screening for eligibility criteria and provision of informed consent, or assent for minors. Participants were followed prospectively through biannual household visits (‘survey-based population’; active surveillance), and at visits to local study health facilities, as-needed, for presentation of fever or other malaria symptoms (“clinic-based subpopulation”; symptomatic passive surveillance) (Fig. 6 ). Three local health facilities were included in our study, one per health area. The chosen facility was the main government clinic in two of these health areas (Bu – rural, Kimpoko – peri-urban). In urban Voix de Peuple, one private clinic was selected due to the diverse patient population it served. Only households within the clinic catchment areas that were located within 5 km from the clinic were eligible for the study. Fig. 6: Study design overview [51] . Biannual household study visits occurred at baseline and three follow-ups over a 20-month longitudinal period in which household demographics and individual health surveys were collected, malaria RDTs were performed, and DBS were collected. Participants who developed fever or other malaria symptoms during follow-up visited study health clinics, where clinical questionnaires, malaria RDTs, a DBS, and hemoglobin testing were performed. Study participants completing household surveys were included in the survey population; those who also visited the clinic at least once for malaria symptoms were included in the clinic subpopulation. DBS dried blood spot, RDT rapid diagnostic test. Full size image Household surveys were conducted between February 2015 and October 2016 (20 months of active surveillance), with baseline and second follow-up surveys largely occurring during the rainy season, and first and third (final) follow-up surveys occurring during the dry season. Symptomatic clinic visits continued beyond the completion of household surveys, through December 2017, for 34 months of passive surveillance. At baseline and follow-up surveys, household-level and individual-level questionnaires were collected to ascertain demographic information, household characteristics (e.g., housing materials, possessions for wealth indicators, bed net ownership and use), health status and clinical data (e.g., malaria diagnostic history, recent symptoms, treatment use). All participants were screened for malaria infection at each visit using a combination RDT detecting P. falciparum -specific HRP2 and pan- Plasmodium LDH) antigens (SD Bioline Ag P.f./Pan RDT [05FK60], Alere, Gyeonggi-do, Republic of Korea). Those positive by RDT (defined as a positive result for either antigen) were referred to study clinics for antimalarial treatment. DBS samples were also collected from all consenting participants at each visit using Whatman 3MM filter paper (Fisher Scientific, Fair Lawn, NJ USA), and were stored with desiccant at -20 °C for future molecular testing. Brief clinical questionnaires were collected from participants at each symptomatic clinic visit throughout the study, alongside malaria RDTs, DBS samples, and hemoglobin testing. Participants were treated at health facilities according to local clinical judgment, as needed, including artemisinin-based combination therapy (ACT) for malaria infection, or referral for blood transfusion if severely anemic. Plasmodium species determination Samples underwent molecular testing at the University of North Carolina Chapel Hill to distinguish Plasmodium species. DNA was extracted from DBS samples using Chelex and saponin [41] . P. falciparum parasitemia was identified using a quantitative real-time duplex PCR assay targeting the LDH and human β-tubulin genes, as previously described [40] , [41] , [42] . We tested samples for P. malariae and P. ovale spp. 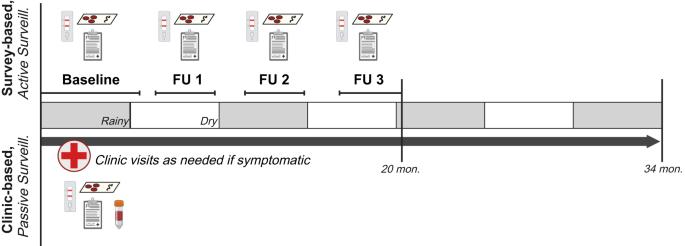Fig. 6: Study design overview51. Biannual household study visits occurred at baseline and three follow-ups over a 20-month longitudinal period in which household demographics and individual health surveys were collected, malaria RDTs were performed, and DBS were collected. Participants who developed fever or other malaria symptoms during follow-up visited study health clinics, where clinical questionnaires, malaria RDTs, a DBS, and hemoglobin testing were performed. Study participants completing household surveys were included in the survey population; those who also visited the clinic at least once for malaria symptoms were included in the clinic subpopulation. DBS dried blood spot, RDT rapid diagnostic test. parasitemia using a semi-quantitative, duplex real-time PCR assay targeting the 18S ribosomal subunit (Supplementary Table 6 ) [43] , [44] . A single replicate of non-falciparum PCR assays were run on samples and considered positive if amplification occurred at cycle thresholds (Cts) < 40. P. falciparum samples were run in duplicate and were considered positive if at least one sample amplified at a Ct <38, or both amplified between Cts ≥38 and <40, as previously described [45] . Semi-quantitative P. malariae and P. ovale spp. parasite densities were estimated from standard curves made using serially-diluted 18 S rRNA plasmid DNA (BEI Resources: #MRA-179 and #MRA-180), assuming six plasmid copies per parasite genome [46] . Non-falciparum parasitemias were then multiplied by 4.0 to account for a 4-fold dilution of blood from three DBS punches [47] , improving comparability with P. falciparum parasitemia quantification. DNA samples with evidence of dehydration were rehydrated prior to PCR testing using 50 µL of molecular-grade water; rehydrated samples were excluded from parasite density analyses. Negative (water) controls were included on all PCR runs. P. vivax was not tested in this study as previously published estimates of P. vivax prevalence in Kinshasa Province from a similar time period (2013-14) indicated low prevalence in the region (0 to <2%) [30] . Population All participants with a baseline DBS available for testing were included in the study. The Kinshasa longitudinal cohort study population provided two distinct types of data utilized in this study: (1) The “survey-based” analysis consists of participant survey data and clinical samples collected at active surveillance household visits for all those enrolled at baseline, and (2) the “clinic-based” analysis consists of participant clinical survey data and samples collected from the subset of the survey-based population who had samples collected at the baseline household enrollment visit, and who visited study clinics as-needed when symptomatic during follow-up (passive surveillance). Samples derived from all study touchpoints (household surveys + clinic visits) were combined to estimate overall infection burden, and also stratified by population type (survey vs. clinic) to account for differences between their predominantly asymptomatic vs. symptomatic natures. Characteristics between the broader survey population and the nested clinic subpopulation were assessed (Supplementary Table 1 ). Weighting was not performed as factors driving selection into the clinic subpopulation were expected to be directly related to the probability of the outcome. Data analysis The primary outcomes in this study were P. malariae, P. ovale spp., and P. falciparum infection confirmed by real-time PCR. Demographic and clinical characteristics were summarized by Plasmodium species across study populations, and the incidence and prevalence of infections were estimated across the 34-month study follow-up period. Parasite densities were descriptively summarized by species and infection type (mixed vs. single-species). Cumulative incidences of first P. malariae, P. ovale spp., and P. falciparum infections were calculated using Kaplan-Meier methods among participants who were PCR-negative at baseline for the Plasmodium species of interest. Incidences were estimated as the inverse of the survival function, measuring time (in months) to the first detected infection since baseline. Participants in the survey population were censored at the time of their last study household visit. Participants in the clinic subpopulation were censored at the end of passive surveillance follow-up, as participants were eligible to continue visiting study health clinics even after the final active follow-up, if symptomatic. Similarly, in the total population, participants who were lost to follow-up prior to the final household survey and had never visited study clinics during follow-up were censored at the time of their last study household visit. Otherwise, those in the total population who completed the final household follow-up were censored at the end of the full study period. Participants dropped out of the at-risk population at the time of their first infection event. We assumed no competing risks for malaria infection since infection by one species would not preclude infection by another, and measured mortality events in the study were low ( n = 26). Demographic characteristics associated with incidence of first infection were evaluated by log-rank testing of stratified cumulative incidence curves. Prevalences of P. malariae, P. ovale spp., and P. falciparum were estimated overall and by species across follow-up. Factors associated with non-falciparum infection prevalences were evaluated using crude linear binomial generalized estimating equation (GEE) models accounting for repeated testing of participants over time. Possible factors associated with malaria infection were modeled individually. An exchangeable working correlation matrix was assumed for GEE models, and robust standard errors were estimated for calculation of 95% confidence intervals (CIs). While three-level clustering of participants nested within households, and households within village sites is present in the study, this clustering structure was too complex to account for using mixed-effect modeling because of the low number of P. malariae and P. ovale outcomes detected in this study. Therefore, the GEE model was used. We also assessed the frequency of multiple same-species non-falciparum infections detected within a participant throughout follow-up; however, these were not distinguished between acute reinfection events, or chronic carriage of a prior infection. Household wealth was computed through adaptation of the Demographic and Health Survey method and categorized into quintiles as previously described , [48] . Quintiles were collapsed into three categories for analysis, and wealth at baseline was carried forward for all subsequent study visits. Seasonality was defined by month, classifying October through April as the rainy season. Anemia severity at symptomatic clinic visits was classified according to hemoglobin (Hb) level, following WHO categories for age-, sex-, and pregnancy-specific cut-points [49] ; severe anemia was defined as Hb<7.0 g/dL for children <5 years, and Hb <8.0 g/dL for all others. Cases were categorized as any anemia vs. no anemia, and comparing moderate/severe vs. mild/no anemia cases. Fever was defined as an axillary temperature >37.5 °C as measured at symptomatic clinic visits, or as self-reported fever within the prior week at baseline and follow-up surveys. Missing data were summarized and excluded from statistical analyses. Dataset construction and cleaning were performed using SAS (version 9.4), and analyses were conducted in R (version 4.0.2) primarily using tidycmprsk, ggsurvfit , and gee packages. The full list of R packages used in analysis is listed in Supplemental Table 7 . Chi-square and Fisher’s Exact tests were performed for statistical comparison of categorical variables. Kruskal-Wallis rank sum tests were performed for comparison of continuous variables, including parasite density distributions across species, assuming nonnormality. All p -values were two-sided. Informed consent, and assent where required, was obtained from all participants or their legal guardians prior to study enrollment and sampling. The study was approved by the Institutional Review Boards at the University of North Carolina at Chapel Hill (IRB#: 14-0489) the University of Iowa (#201701201), and the Kinshasa School of Public Health (ESP/CE/015/014). Reporting summary Further information on research design is available in the Nature Portfolio Reporting Summary linked to this article.